In vivocapture and label-free detection of early metastatic cells Breast cancer is a leading cause of death for women, with mortality resulting from metastasis. Metastases are often detected once tumour cells affect the function of solid organs, with a high disease burden limiting effective treatment. Here we report a method for the early detection of metastasis using an implanted scaffold to recruit and capture metastatic cells in vivo , which achieves high cell densities and reduces the tumour burden within solid organs 10-fold. Recruitment is associated with infiltration of immune cells, which include Gr1 hi CD11b + cells. We identify metastatic cells in the scaffold through a label-free detection system using inverse spectroscopic optical coherence tomography, which identifies changes to nanoscale tissue architecture associated with the presence of tumour cells. For patients at risk of recurrence, scaffold implantation following completion of primary therapy has the potential to identify metastatic disease at the earliest stage, enabling initiation of therapy while the disease burden is low. The discovery of metastatic spread of a primary tumour is often associated with poor prognosis, owing to the fact that metastases typically go undetected until the function of one or more organs have been affected. Identification of metastasis before significant organ invasion would enable interventional strategies to halt disease progression while the disease burden is still low [1] . Much attention has been focused on screening for the presence of circulating tumour cells (CTCs) as a measure of metastasis. CTCs are present at low numbers in the blood and technologies such as microfluidic devices have been designed to capture and quantify the number of CTCs from patient blood samples [2] , [3] . Recently, a system that also enables expansion of CTCs following capture has been developed [4] . These technologies provide opportunities for studying the biology of CTCs, development of biomarkers, disease monitoring and personalized medicine strategies. However, CTCs can remain in the circulation for long periods of time before homing to and colonizing a metastatic site, with some tumour cells being shed at early points during tumour progression [5] , [6] . Thus, we sought to develop a method for capturing and detecting cells that have extravasated and colonized a site, which are steps in the metastatic cascade downstream from the circulation of tumour cells. Paget’s seed-and-soil hypothesis, developed a century ago, proposed that dissemination of cancer cells to specific sites in the body, such as lung or liver, is not random but rather is due to the receptive microenvironments at those sites [7] . More recently, studies have shown that before colonization of a metastatic site, a ‘pre-metastatic niche’ is established by VEGFR1+ bone marrow-derived hematopoietic progenitor cells [8] . These cells create a tumour-supportive microenvironment comprised of several cell types, including hematopoietic and endothelial progenitor cells and immune cells that condition the environment with matrix proteins, cytokines and chemokines to facilitate migration, invasion, proliferation and angiogenesis at the metastatic site [9] , [10] , [11] . Immune cells, in particular, play critical roles in homing and colonization of the metastatic site. Macrophages facilitate extravasation of metastatic cells as they begin the process of colonization [12] . Myeloid-derived suppressor cells [13] , [14] , [15] and inflammatory monocytes [16] have also been associated with metastatic sites, and neutrophils have been shown to facilitate transendothelial migration of tumour cells. Importantly, the existence of the pre-metastatic niche indicates that a site could be engineered to recapitulate the microenvironment of the niche in vivo . In this report, we develop a biomaterial implant to recruit and capture metastatic cells, combined with an imaging system using inverse spectroscopic optical coherence tomography (ISOCT) for label-free detection of cancer cells at the implant, that together constitute a system to detect early metastases. The implants are microporous scaffolds composed of poly(lactide-co-glycolide) (PLG), a material that is FDA approved for a variety of applications. We also investigate if the capture of extravasating metastatic cells can reduce colonization of solid organs and consequently tumour burden, which could have therapeutic implications. In addition, modulation of the local immune environment may be a versatile approach for recruiting tumour cells that is distinct from strategies that mimic the microenvironment of a target organ, such as bone [17] , [18] . To this end, the immune response at the implant, which consists of numerous cell types such as macrophages and neutrophils, is hypothesized to mediate recruitment of tumour cells [8] , [10] , [12] , [16] , [19] , [20] , and this mechanism of recruitment is investigated through localized delivery of the chemokine CCL22 and transplantation of myeloid-derived suppressor cells. Recruited tumour-associated myeloid-derived suppressor cells, in part, contribute to the formation a pre-metastatic niche, which supports a permissive environment for the capture of tumour cells in the scaffold. This approach for immune cell-mediated capture and early detection of metastatic cells has the potential to be broadly applicable to many types of cancer. Scaffolds for in vivo capture of metastasizing cells An orthotopic model of human breast cancer metastasis was employed to investigate the capture of metastatic cells at a biomaterial implant. tdTomato- and luciferase-expressing MDA-MB-231BR (231BR) cells, a highly metastatic variant of the MDA-MB-231 cell line [21] , were transplanted into the right mammary fat pads of female NOD/SCID-IL2Rγ −/− (NSG) mice ( Fig. 1c ). One week after tumour inoculation, microporous PLG scaffolds (5-mm diameter, 2-mm height, Supplementary Fig. 1a–c ) were implanted into the peritoneal fat pads, a site to which 231BR cells are not reported to colonize, yet supports the vascularization of PLG scaffolds. Bioluminescence imaging and histological analysis of peritoneal fat pads removed 28 days after tumour inoculation demonstrated the presence of tumour cells within the implanted PLG scaffold ( Fig. 1a,d ) and the absence of tumour cells in fat pads without scaffolds ( Fig. 1b,e ), indicating that the local environment generated by implantation of the scaffold enabled recruitment of metastatic cells. Primary tumour growth was not affected by either implantation of scaffolds or a mock surgery ( Supplementary Fig. 2 ). Staining for fibronectin, a matrix protein reported to be involved in establishment of the pre-metastatic niche [8] , indicated that fibronectin was present in scaffolds implanted in both healthy and tumour-bearing mice as early as 7 days post implantation ( Supplementary Fig. 1d ). Interestingly, recruitment of cells to the scaffold was not site-specific, as tumour cells were detected in scaffolds implanted in the subcutaneous tissue ( Supplementary Fig. 3 ). 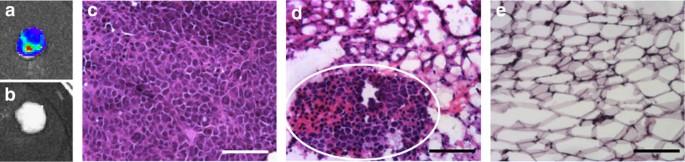Figure 1: PLG scaffolds recruit metastatic tumour cells. Tissues were isolated at day 28 post-tumour inoculation (21 days after scaffold implantation or mock surgery). (a,b) Bioluminescence imaging (BLI) of peritoneal fat pads receiving scaffold implants (a) or mock surgeries (b). (c-e) Hematoxylin and eosin (H&E) staining of the primary tumour (c) a fat pad containing a scaffold (white circle indicates metastatic cluster) (d) and a fat pad without a scaffold (e). Scale bars, 100 μm. Figure 1: PLG scaffolds recruit metastatic tumour cells. Tissues were isolated at day 28 post-tumour inoculation (21 days after scaffold implantation or mock surgery). ( a , b ) Bioluminescence imaging (BLI) of peritoneal fat pads receiving scaffold implants ( a ) or mock surgeries ( b ). ( c - e ) Hematoxylin and eosin (H&E) staining of the primary tumour ( c ) a fat pad containing a scaffold (white circle indicates metastatic cluster) ( d ) and a fat pad without a scaffold ( e ). Scale bars, 100 μm. Full size image Scaffolds reduce tumour burden in solid organs We subsequently investigated whether capturing tumour cells in scaffolds would reduce colonization of standard metastatic sites, such as the lung and liver. At 28 days post-tumour inoculation, the relative abundance of tumour cells, reported as the ratio of tdTomato-positive tumour cells to total cells, was determined. For mice that received scaffolds, the relative abundance of tumour cells in the lung was 1:5,400, compared with 1:645 for mice receiving a mock surgery ( Fig. 2a , Supplementary Fig. 4 ). Thus, the presence of a scaffold reduced the tumour burden for the lung by 88±7% (average±s.e.m.). Histological analysis of lung sections confirmed a reduction in the tumour cell burden with scaffold implantation ( Fig. 2b,c ), with an average of 1.7±0.5 metastatic lesions per section observed in the lungs of scaffold-bearing mice, compared with 5.5±1.7 lesions per section in mice receiving mock surgeries. Furthermore, flow cytometric analysis of cells isolated from the liver showed detectable tumour cells in eight out of eight mice receiving mock surgeries, while mice receiving scaffold implants only exhibited detectable tumour cells in two of eight livers ( P <0.01, Fisher’s exact test). 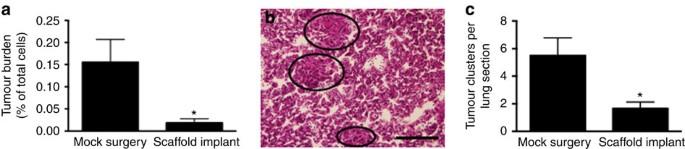Figure 2: Recruitment of tumour cells to scaffolds reduces tumour burden in lung. (a) Flow cytometric analysis of the percentage of tdTomato-positive tumour cells in cells isolated from lungs at day 28 post-tumour inoculation. Data shown as mean±s.e.m. (n=8, 2 independent biological replicates). *P<0.01 compared with mock surgery (Mann–Whitney test). (b) H&E staining of lung section (black circles indicate metastatic clusters). Scale bar, 200 μm. (c) Histological analysis of H&E-stained lung sections to determine the number of tumour clusters per section. Data shown as mean±s.e.m. (n=12, 2 independent biological replicates). *P<0.05 compared with mock surgery (Mann–Whitney test). Figure 2: Recruitment of tumour cells to scaffolds reduces tumour burden in lung. ( a ) Flow cytometric analysis of the percentage of tdTomato-positive tumour cells in cells isolated from lungs at day 28 post-tumour inoculation. Data shown as mean±s.e.m. ( n =8, 2 independent biological replicates). * P <0.01 compared with mock surgery (Mann–Whitney test). ( b ) H&E staining of lung section (black circles indicate metastatic clusters). Scale bar, 200 μm. ( c ) Histological analysis of H&E-stained lung sections to determine the number of tumour clusters per section. Data shown as mean±s.e.m. ( n =12, 2 independent biological replicates). * P <0.05 compared with mock surgery (Mann–Whitney test). Full size image Early detection of tumour cells in scaffold The potential to use scaffolds for early detection of metastasis was determined by quantifying the percentage of tumour cells in intraperitoneal and subcutaneous scaffolds compared with the lung and liver at day 14 post-tumour inoculation. In a group of eight mice, most intraperitoneal scaffolds (15/16) contained tumour cells at this time point, while none of the mice had detectable tumour cells in the lung and liver ( Fig. 3a ). In a separate group of mice, all subcutaneous scaffolds (10/10) contained tumour cells. The incidence of detectable metastatic disease at this early time point was lower than at day 28 post-tumour inoculation. At day 28 post-tumour inoculation in scaffold-bearing mice, the lung and liver exhibited tumour cells in 8 and 2 of the eight mice, respectively. Furthermore, for mice receiving mock surgeries instead of scaffold implants, the incidence of metastatic cells in both the lung and liver increased to eight out of eight mice. Importantly, at day 14 post inoculation, while none of the lungs and livers exhibited detectable tumour cells, both intraperitoneal and subcutaneous scaffolds had a detectable percentage of tumour cells (0.019±0.005% for intraperitoneal scaffolds and 0.044±0.017% for subcutaneous scaffolds) ( Fig. 3b , Supplementary Fig. 5 ). This ability to detect tumour cells in the scaffold before detection in the lungs and liver may enable the early detection of metastatic disease through imaging the scaffold. 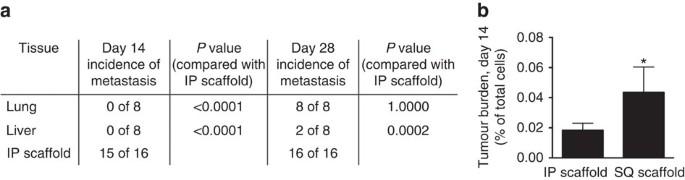Figure 3: Early detection of tumour cells in scaffolds. Flow cytometric analysis of tdTomato-positive tumour cells in tissues isolated from mice at day 14 and 28 post-tumour inoculation. (a) Number of mice with tumour cells detectable in each tissue in a group of 8 mice at day 14 or 28 post-tumour inoculation. Each mouse received two intraperitoneal (IP) scaffolds.Pvalues from Fisher’s exact test. (b) Percentage of tdTomato-positive cells in the total cell population isolated from IP scaffolds and subcutaneous (SQ) scaffolds at day 14 post-tumour inoculation. Data shown as mean±s.e.m. (n=16 for IP scaffold,n=10 for SQ scaffold, two independent biological replicates). *P<0.05 compared with IP scaffold (Mann–Whitney test). Figure 3: Early detection of tumour cells in scaffolds. Flow cytometric analysis of tdTomato-positive tumour cells in tissues isolated from mice at day 14 and 28 post-tumour inoculation. ( a ) Number of mice with tumour cells detectable in each tissue in a group of 8 mice at day 14 or 28 post-tumour inoculation. Each mouse received two intraperitoneal (IP) scaffolds. P values from Fisher’s exact test. ( b ) Percentage of tdTomato-positive cells in the total cell population isolated from IP scaffolds and subcutaneous (SQ) scaffolds at day 14 post-tumour inoculation. Data shown as mean±s.e.m. ( n =16 for IP scaffold, n =10 for SQ scaffold, two independent biological replicates). * P <0.05 compared with IP scaffold (Mann–Whitney test). Full size image Label-free detection of metastasis at the scaffold ISOCT [22] was applied to directly visualize the scaffold architecture and provide quantitative measurement of the ultrastructural changes induced by the cancer cells. ISOCT is a light scattering-based technique capable of non-invasive three-dimensional (3D) imaging of tissue morphology with micron-level resolution and millimeter-level penetration depth [23] , [24] . In addition, for each 3D resolution voxel (15 × 15 × 2 μm) ISOCT also performs a spectroscopic analysis and quantifies the power of the spectra by a scattering model I ( λ ) ∝ λ D-4 22 . D is the shape factor that physically defines the macromolecular density correlation function for a range of length scales from ∼ 40 to 350 nm (ref. 25 ), with higher D values indicating a more clumped structure. It has been demonstrated that D is a ubiquitous marker of the ultrastructural alterations in the early stages of various cancer types despite their different etiologies [26] , [27] , [28] , [29] , [30] , with both neoplastic cells and the surrounding stroma exhibiting an increase in D in part due to chromatin condensation and collagen remodelling, respectively [27] , [30] , [31] . Given the nanoscale sensitivity of measuring D and the tissue-level imaging capability, we hypothesized that ISOCT could be an effective approach for detection of cancer cells within the scaffold. In vitro studies were performed to demonstrate that ISOCT could capture changes in D for cells and matrices, and the technique was subsequently applied to in situ imaging of scaffolds. ISOCT analysis of 231BR cell pellets confirmed that they had a higher D than normal mammary epithelial cells (MCF10A) and cells isolated from lungs of tumour-free NSG mice (3.49±0.12, 2.74±0.15 and 3.00±0.13, respectively, Supplementary Fig. 6a ). Changes to collagen remodelling by 231BR cells were evaluated by culturing 231BR cells in collagen gels for 3 days, after which cells were extracted and the gels were analysed using ISOCT. 231BR-conditioned matrices exhibited a D value of 1.69±0.08 compared with a D value of 1.29±0.04 for gels cultured with media ( Supplementary Fig. 6b ). With confirmation of the technique in vitro , in situ ISOCT analysis was applied to scaffolds, which demonstrated that scaffolds implanted in the subcutaneous tissue of tumour-bearing mice also had an increase in D at day 14 post-tumour inoculation compared with control scaffolds in tumour-free mice ( Fig. 4 ), with an average D value of 5.77±0.38 in tumour-bearing mice compared with 4.71±0.17 in tumour-free mice. This increase in D is consistent with the changes associated with the presence of cancerous cells and the ensuing reorganization of the extracellular matrix. These results indicate that this method can be used for label-free detection of micrometastases within the scaffold at the early stages of metastatic disease. 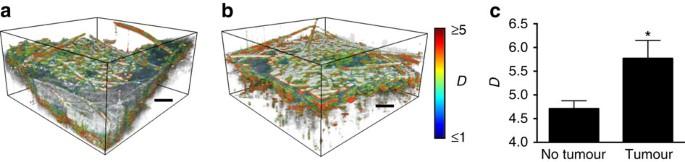Figure 4: Detection of tumour cells in scaffold using ISOCT. (a,b) Representative 3D maps ofDgenerated fromin situISOCT analysis of subcutaneous scaffolds implanted in tumour-free (a) and tumour-bearing (b) mice at day 14 post-tumour inoculation. Scale bars, 200 μm. (c) AverageDvalue for subcutaneous scaffolds in tumour-free (‘No Tumor’) and tumour-bearing (‘Tumor’) mice. Data shown as mean±s.e.m. (n=6, 2 independent biological replicates). *P<0.05 compared with tumour-free mice (Mann–Whitney test). Figure 4: Detection of tumour cells in scaffold using ISOCT. ( a , b ) Representative 3D maps of D generated from in situ ISOCT analysis of subcutaneous scaffolds implanted in tumour-free ( a ) and tumour-bearing ( b ) mice at day 14 post-tumour inoculation. Scale bars, 200 μm. ( c ) Average D value for subcutaneous scaffolds in tumour-free (‘No Tumor’) and tumour-bearing (‘Tumor’) mice. Data shown as mean±s.e.m. ( n =6, 2 independent biological replicates). * P <0.05 compared with tumour-free mice (Mann–Whitney test). Full size image Immune cells contribute to tumour cell recruitment Given the critical role of various immune cells types in establishing the pre-metastatic niche [8] , [10] , [12] , [16] , [19] , [20] , we hypothesized that the immune response to the scaffold was mediating recruitment of tumour cells. For analysis of the immune environment within the scaffolds, we used an immune-competent mouse model in addition to the NSG model to account for effects of both the innate and adaptive immune response. Scaffolds implanted into BALB/c mice inoculated with 4T1 mouse breast cancer cells also demonstrated metastatic cells within the scaffold, indicating that the scaffold could still achieve homing within the context of an intact immune system ( Supplementary Fig. 7 ). Inflammatory cells proposed to be involved in recruiting tumour cells were characterized within the peritoneal fat pads of mice in the presence and absence of a scaffold. A high density of CD45-positive leukocytes was present in histological sections of the scaffold, with no observed CD45-positive leukocytes present in fat pads of mice receiving mock surgeries ( Fig. 5a,b ). The ability of CD45-positive leukocytes to influence homing of tumour cells was investigated through migration assays using media conditioned by splenocytes isolated from spleens of tumour-bearing mice, as the spleen contains a large number of immune cells and has a distribution of immune cells similar to the scaffolds, with the predominant cell type being Gr1 hi CD11b + cells ( Supplementary Fig. 8 ). Migration of both cell types was significantly increased in the presence of splenocyte-conditioned media relative to unconditioned media ( Fig. 5c,d ), with 261±35 migrating 231BR cells per well in conditioned media compared with 137±20 cells in unconditioned media and 521±22 migrating 4T1 cells per well in conditioned media compared with 292±23 cells in unconditioned media. These results indicate that paracrine signalling from immune cell populations similar to those present in the scaffold can induce migration of tumour cells. 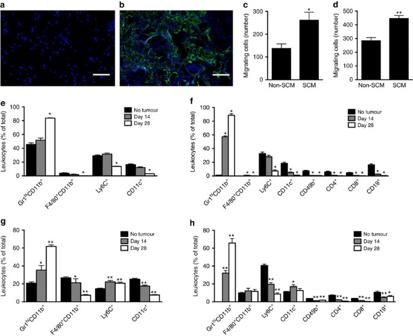Figure 5: Evaluation of the immune environment within scaffolds. (a,b) CD45 immunolabeling (green) at day 28 post-tumour inoculation of fat pads receiving mock surgery (a) or scaffold implant (b). Nuclei are blue. Scale bar, 100 μm. (c,d) Number of migrating 231BR (c) or 4T1 (d) cells in the presence of splenocyte-conditioned media (SCM) or non-conditioned media (non-SCM). Data shown as mean±s.e.m. (n=6, 2 independent biological replicates). *P<0.05 and **P<0.005 compared with non-conditioned media (Mann–Whitney test). (e–h) Flow cytometric analysis of cells removed from lungs (e,f) and scaffolds (g,h) of tumour-free and tumour-bearing (day 14 and 28) NSG (e,g) or BALB/c (f,h) mice. The model used for mice with tumours involved the inoculation of tumour cells at day 0, with scaffolds implanted at day 7. The evaluation of scaffolds in tumour-free mice was performed on day 7 post implantation. Cell populations are reported as percentage of total CD45-positive leukocytes. Data shown as mean±s.e.m. (n=5 for lungs,n=10 for scaffolds, 2 independent biological replicates). *P<0.05 and **P<0.005 compared with no tumour (Mann–Whitney test). Figure 5: Evaluation of the immune environment within scaffolds. ( a , b ) CD45 immunolabeling (green) at day 28 post-tumour inoculation of fat pads receiving mock surgery ( a ) or scaffold implant ( b ). Nuclei are blue. Scale bar, 100 μm. ( c,d ) Number of migrating 231BR ( c ) or 4T1 ( d ) cells in the presence of splenocyte-conditioned media (SCM) or non-conditioned media (non-SCM). Data shown as mean±s.e.m. ( n =6, 2 independent biological replicates). * P <0.05 and ** P <0.005 compared with non-conditioned media (Mann–Whitney test). ( e – h ) Flow cytometric analysis of cells removed from lungs ( e , f ) and scaffolds ( g , h ) of tumour-free and tumour-bearing (day 14 and 28) NSG ( e , g ) or BALB/c ( f , h ) mice. The model used for mice with tumours involved the inoculation of tumour cells at day 0, with scaffolds implanted at day 7. The evaluation of scaffolds in tumour-free mice was performed on day 7 post implantation. Cell populations are reported as percentage of total CD45-positive leukocytes. Data shown as mean±s.e.m. ( n =5 for lungs, n =10 for scaffolds, 2 independent biological replicates). * P <0.05 and ** P <0.005 compared with no tumour (Mann–Whitney test). Full size image Before and after the introduction of cancer cells, we analysed the local immune environment of the implanted scaffold, which was compared with that of the lung, a common site of breast cancer metastasis. Flow cytometric analysis demonstrated that during disease progression, the most notable change in the relative distribution of immune cells was an increase in Gr1 hi CD11b + cells ( Fig. 5e–h , Supplementary Figs 9–11 ). This increase was consistent in both the NSG and BALB/c mouse models, and was found in both the lungs and scaffolds. In the lungs of the NSG mice, the percentage of Gr1 hi CD11b + cells increased from 45±2% at day 0 (no tumour) to 52±3% at day 14 post-tumour inoculation, to 84±1% at day 28 post-tumour inoculation ( Fig. 5e ). Following this trend, the percentage of Gr1 hi CD11b + cells found in the scaffolds from the NSG mice increased from 21±1% (tumour-free mice), to 35±5% at day 14 post-tumour inoculation, to 62±2% at day 28 post-tumour inoculation ( Fig. 5g ). In the lungs of BALB/c mice, Gr1 hi CD11b + cells increased from 1±0.1% at day 0 (tumour-free mice) to 57±1% at day 14 post-tumour inoculation, to 89±2% at day 28 post-tumour inoculation ( Fig. 5f ). Likewise, within the scaffolds from the BALB/c mice, Gr1 hi CD11b + cells increased from 0.1±0.01% (no tumour) to 32±3% at day 14 post-tumour inoculation, to 66±5% at day 28 post-tumour inoculation ( Fig. 5h ). These results highlight the correlation between disease exposure time and the relative abundance of Gr1 hi CD11b + cells found in both the lungs and scaffolds of affected animals, and show that the immune environment within a metastatic organ site is similar to that of an implanted scaffold. We subsequently investigated the hypothesis that modulation of the inflammatory microenvironment within the scaffold site would influence recruitment of metastatic cells. Lentiviral vectors were delivered from the scaffold to promote localized transgene expression for the duration of the study ( Supplementary Fig. 12 ). The chemokine CCL22 was selected for expression as it induces migration of splenocytes harvested from NSG mice ( Supplementary Fig. 13a ) yet does not influence the migration of tumour cells ( Supplementary Fig. 13b ). Flow cytometric analysis of CCL22 scaffolds at day 7 post implantation indicated an increase in Gr1 hi CD11b + cells, which have been implicated in the pre-metastatic niche [10] , [14] , [15] , from 20±2% to 29±3% in NSG mice and from 14±1% to 19±1% in BALB/c mice ( Fig. 6a,c ). In addition, F4/80 + CD11b + inflammatory macrophages, which are recruited to circulating metastatic cells as they undergo extravasation and begin colonization [12] , increased from 28±2% to 34±2% in the NSG model and from 10±1% to 14±1% in the BALB/c model ( Fig. 6a,c ). Furthermore, CCL22 expression increased the number of tdTomato-positive tumour cells present in the scaffold in both mouse models at day 7 post implantation (day 14 post-tumour inoculation), with an average of 92±16 cells compared with an average of 23±4 cells for β-galactosidase expression in NSG mice and an average of 62±5 cells compared with an average of 20±2 cells for β-galactosidase expression in BALB/c mice ( Fig. 6b,d ). 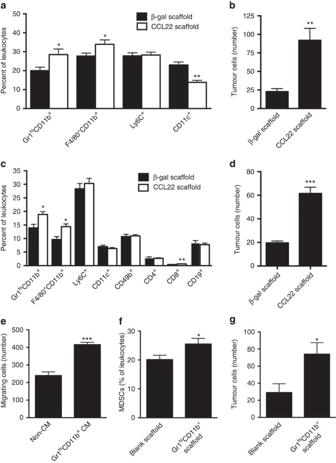Figure 6: Immunomodulation of the scaffold microenvironment influences recruitment of tumour cells. Flow cytometric analysis at day 14 post-tumour inoculation of cells removed from scaffolds containing a CCL22 or β-galactosidase (control) vector implanted in NSG (a,b) or BALB/c (c,d) mice. Cell populations are reported as percentage of total CD45-positive leukocytes (a,c) or total number of tumour cells in the scaffold (b,d). Data shown as mean±s.e.m. (n=10, 2 independent biological replicates). *P<0.05, **P<0.005 and ***P<0.001 compared with β-galactosidase scaffolds (Mann–Whitney test). (e) Number of migrating 231BR cells in the presence of Gr1hiCD11b+cell-conditioned media (Gr1hiCD11b+CM) or non-conditioned media (non-SCM). Data shown as mean±s.e.m. (n=6, 2 independent biological replicates). ***P<0.001 compared with non-conditioned media (Mann–Whitney test). (f,g) Flow cytometric analysis at day 14 post-tumour inoculation of cells removed from blank scaffolds or scaffolds seeded with Gr1hiCD11b+cells. Cell populations are reported as the percentage of Gr1hiCD11b+cells in the total leukocyte population (f) or total number of tumour cells in the scaffold (g). Data shown as mean±s.e.m. (n=10, 2 independent biological replicates). *P<0.05 compared with blank scaffold (Mann–Whitney test). Figure 6: Immunomodulation of the scaffold microenvironment influences recruitment of tumour cells. Flow cytometric analysis at day 14 post-tumour inoculation of cells removed from scaffolds containing a CCL22 or β-galactosidase (control) vector implanted in NSG ( a , b ) or BALB/c ( c , d ) mice. Cell populations are reported as percentage of total CD45-positive leukocytes ( a , c ) or total number of tumour cells in the scaffold ( b , d ). Data shown as mean±s.e.m. ( n =10, 2 independent biological replicates). * P <0.05, ** P <0.005 and *** P <0.001 compared with β-galactosidase scaffolds (Mann–Whitney test). ( e ) Number of migrating 231BR cells in the presence of Gr1 hi CD11b + cell-conditioned media (Gr1 hi CD11b + CM) or non-conditioned media (non-SCM). Data shown as mean±s.e.m. ( n =6, 2 independent biological replicates). *** P <0.001 compared with non-conditioned media (Mann–Whitney test). ( f , g ) Flow cytometric analysis at day 14 post-tumour inoculation of cells removed from blank scaffolds or scaffolds seeded with Gr1 hi CD11b + cells. Cell populations are reported as the percentage of Gr1 hi CD11b + cells in the total leukocyte population ( f ) or total number of tumour cells in the scaffold ( g ). Data shown as mean±s.e.m. ( n =10, 2 independent biological replicates). * P <0.05 compared with blank scaffold (Mann–Whitney test). Full size image A cell population upregulated by CCL22 delivery, Gr1 hi CD11b + cells, was next transplanted on the scaffold to directly modulate the local immune environment and further demonstrate that the immune environment mediates metastatic cell recruitment. Gr1 hi CD11b + cells were selected for these studies given their established role in the pre-metastatic niche, along with migration assays showing soluble factors secreted by Gr1 hi CD11b + cells isolated from spleens of tumour-bearing NSG mice induced migration of 231BR cells ( Fig. 6e ). Interestingly, the Gr1 hi CD11b + cells induced migration to a greater extent than splenocyte-conditioned media ( Supplementary Fig. 14 ). Implantation of scaffolds seeded with Gr1 hi CD11b + cells significantly increased the percentage of Gr1 hi CD11b + cells in the total leukocyte population (from 20±2 to 26±2%, Fig. 6f ) as well as the number of tumour cells (from 29±10 to 74±13 cells, Fig. 6g ) present per scaffold, indicating that Gr1 hi CD11b + cells contributed to recruitment of tumour cells to the scaffold. This study demonstrates a platform technology for the capture and label-free detection of cancer cells early in the onset of the metastatic process. Biomaterial scaffolds were engineered to recruit metastatic cells in vivo through modulation of the local immune environment, with detection of cancer cells based on the tissue nanoarchitecture by ISOCT. The ability of the scaffolds to reduce tumour burden in host organs that are standard sites of breast cancer metastasis suggests the potential use of the scaffold as a therapeutic tool, serving as a sink to capture CTCs. As opposed to models that employ tail vein injections to study lung colonization by directly placing large numbers of tumour cells in the bloodstream [32] , the orthotopic model employed in this study more closely mimics the release of metastatic cells from the primary tumour observed in the clinical setting. The ability of the scaffolds to capture a fraction of the metastatic cells early in disease progression and consequently limit colonization to other organ sites is also a distinguishing feature from purely diagnostic approaches, such as the detection of CTCs in blood samples. Furthermore, cancer cells can be retrieved from scaffolds and analysed for biomarkers unique to the metastatic setting, and targeted therapies could then be developed that are appropriately tailored to metastatic cancer cell biology. The approach of designing scaffolds to capture circulating cells in vivo has been used for cancer as well as regenerative medicine applications. Strategies to develop biomaterial implants that capture endothelial progenitor cells and smooth muscle progenitor cells from the bloodstream have been implemented to promote vascularization of the implant [33] , [34] , [35] . In addition, biomaterial scaffolds designed to recruit endogenous stem cells have promoted bone regeneration [36] and cardiac repair [37] . Strategies to capture circulating cancer cells in vivo have focused on mimicking the microenvironment of a target organ, as demonstrated by the use of scaffolds that mimic the bone microenvironment for capture of breast cancer cells [18] and hematopoietic cancer cells [17] . This technology used a broader approach of recruiting metastasizing breast cancer cells through local immune modulation, as immune cells have been shown to play critical roles in recruiting metastatic cells [9] , [10] , [12] , [14] , [15] , [16] , [19] . Given the importance of immune cells in regulating metastasis for several cancers, this approach may provide a more versatile method for capture of extravasating cancer cells in vivo . Further, the coupling of cell capture strategies with label-free imaging methods (that is, ISOCT) demonstrates the potential for using this approach as a diagnostic tool. These scaffolds also provide an enabling tool to control the cell types and signals present at a local site to identify regulators of early events in colonization, which could lead to novel therapeutic targets for prevention of metastasis. The microenvironment within the scaffolds can be modified through cell transplantation, presentation of extracellular matrix proteins, or delivery of proteins or gene therapy vectors [38] , [39] , [40] , [41] and represents a platform for molecularly dissecting the biological cues that underlie the recruitment of metastatic cells. Herein Gr1 hi CD11b + cells were either recruited through chemokine expression or transplanted on the scaffold, which enhanced recruitment of extravasating tumour cells. Gr1 hi CD11b + cells accumulate in the spleen during tumour progression [42] , and previous reports indicate they are recruited to a pre-metastatic niche by inflammatory chemokines [43] . While the increase in Gr1 hi CD11b + cells in the scaffold was modest, the increase in cancer cells was substantial, which is consistent with multiple effects of Gr1 hi CD11b + cells on tumour cells [44] . Finally, scaffolds, coupled with ISOCT imaging, functioned as a sensor to detect tumour cells early in the onset of metastatic progression, which could enable therapeutic intervention while the disease burden is low. While whole-body imaging techniques do not provide the requisite sensitivity and resolution to detect a few cells as they colonize a metastatic site, optical imaging is suited for this application. Optical coherence tomography (OCT) conventionally has been used to provide microscopic reconstruction of tissue morphology with a spatial resolution on the order of several microns. Accordingly, OCT has been applied to in vivo imaging of the tumour microenvironment [45] . ISOCT models tissue as a medium with a continuously fluctuating macromolecular mass density [46] . By measuring its optical properties, the mass density correlation function can be inversely recovered at each 3D voxel of spatial resolution [22] . Moreover, because ISOCT uses the spectral information to measure the self-interference within a resolution-limited voxel, the length scale of sensitivity of ISOCT can be as small as ∼ 35nm, far beyond the resolution limit of conventional microscopy [47] , [48] , [49] . While the necessary penetration depth and large volume of a solid organ such as the lung or liver would not be well-suited for ISOCT-based detection of a small number of colonizing cells, the scaffold concentrates metastatic cells in an area beneath the skin, a site that is more readily accessible for imaging. Thus, ISOCT provides a robust approach for identifying the changes to the scaffold microenvironment on colonization by metastatic cells. Taken together, the early detection, reduced burden of metastatic disease and potential to apply targeted therapies afforded by this technology could significantly extend the time to disease progression. Study design The objective of the study was to use biomaterials scaffolds and optical imaging techniques to capture and detect metastasizing breast cancer cells in vivo . We hypothesized that due to the local inflammatory response following implantation, the scaffolds become infiltrated with immune cells conducive to recruiting metastatic cells, and that a light scattering-based imaging method could detect changes to the tissue ultrastructure associated with arrival of the cancer cells. Animal studies were performed with at least two independent replicates of 4–8 female 10–14-week-old mice per group with random assignment. Tissues were analysed at day 14 or 28 post-tumour inoculation, with day 14 being the earliest time point for detecting metastasis and day 28 being the final time point, as the primary tumour reached the maximum allowable size. In vitro experiments had multiple samples that were independently repeated at least two times. Tumour inoculation and volume measurement Animal studies were performed in accordance with institutional guidelines and protocols approved by the Northwestern University Institutional Animal Care and Use Committee. Tumour inoculation was performed by injecting 2 × 10 6 231BR (Northwestern University Developmental Therapeutics Core) or 4T1 (ATCC) cells in a volume of 50 μl PBS (Life Technologies) into the number four right mammary fat pads of 10−14-week-old female NSG or BALB/c mice. NSG mice were purchased from The Jackson Laboratory or bred in house. BALB/c mice were purchased from The Jackson Laboratory. Tumour length and width were measured weekly using digital calipers (VWR) beginning at day 14 post inoculation, and tumour volume was calculated using the formula Volume=(Width 2 × Length)/2. Scaffold fabrication and implantation PLG scaffolds were fabricated as previously described [40] . Briefly, microspheres were prepared by emulsifying a 6% solution of PLG (Lakeshore Biomaterials; 75:25 lactide:glycolide, inherent viscosity=0.76 dl g −l ) in dicholoromethane in 1% poly(vinyl alcohol). Microspheres were washed four times with deionized water to remove residual poly(vinyl alcohol) and lyophilized overnight. Next, microspheres were mixed with 250–425-μm salt particles in a 30:1 ratio and pressed in a steel die at 1,500 psi. The scaffolds were then gas-foamed and salt particles were removed by washing in water for 90 min. Scaffolds were sterilized with 70% ethanol and rinsed with water before drying. Incorporation of a viral vector was performed by incubating 1 × 10 9 viral particles in a volume of 10 μl PBS with the scaffold for 8 min. In these studies, tumours were inoculated at day 0 and scaffolds were implanted in the intraperitoneal fat pads or subcutaneous space at day 7. Virus production The lentiviral vector of interest was co-transfected with the packaging vectors pRSV-Rev, pIVS-VSV-G and pMDL-GagPol [50] into HEK-293T cells grown in DMEM (Sigma) containing 10% fetal bovine serum (Life Technologies) for virus production using Lipofectamine 200 (Life Technologies). After 48 h the supernatant was collected. Viral particles were concentrated using PEG-it (Systems Biosciences) and resuspended in PBS. Virus titre was quantified using the qPCR Lentivirus Titration Kit (Applied Biological Materials) according to the manufacturer’s instructions. Bioluminescence imaging Five minutes before imaging, mice were injected intraperitoneally with D-luciferin (Molecular Imaging Products; 20 mg ml −1 in PBS) at 150 mg kg −1 body weight. For whole-animal imaging, mice were anesthetized with inhaled isoflurane and in vivo luciferase expression was evaluated using the IVIS Spectrum imaging system (Caliper Life Sciences). For imaging of tissues, mice were euthanized 5 min after injection with D-luciferin and tissues were retrieved and imaged using the IVIS Spectrum. Histological analysis and immunohistochemistry Organs and implanted scaffolds were retrieved from mice, rinsed in PBS and then immediately flash-frozen in pre-chilled isopentane. The frozen tissue was then embedded in optimal cutting temperature (OCT; Cardinal Health) compound with 30% sucrose. The lungs were sectioned at 12 μm, and the scaffolds and fat pads were sectioned at 14-μm thick sections using a cryostat (Microm HM 525; Microm International) and stored at −20 °C until staining. To determine the presence of tumour cells, slides were fixed with 4% paraformaldehyde (Sigma) for 10 min and stained with Gill III Hematoxylin (Leica) and Eosin Y (Leica). Blinded scoring of the number of tumour clusters in each tissue section was performed by a pathologist. Two sections were analysed per mouse, and in each of two separate experiments, sections from three mice per group were analysed, for a total of six animals per condition. The sections analysed were non-adjacent and separated by at least 5 mm. For immunohistochemistry, sections were fixed for 12 min in 4% paraformaldehyde and stained with a polyclonal rabbit anti-CD45 primary antibody (1:100, Abcam) followed by a CF633 anti-rabbit secondary antibody (1:500, Sigma) or a polyclonal rabbit anti-fibronectin antibody (1:250, Abcam) followed by an Alexa Fluor 488 anti-rabbit secondary antibody (1:500, Life Technologies). Nuclei were labelled with Hoechst 33250 (1:2,000, Invitrogen). Samples were imaged using a Leica SP5 II laser scanning confocal microscope. Flow cytometry Mice were euthanized and tissues were retrieved, minced with microscissors in a 0.38 mg ml −1 solution of Liberase TL or TM (Roche Applied Science) in Hank’s Balanced Salt Solution (HBSS; Life Technologies) and placed at 37 °C for 20 min. Liberase was neutralized with 0.125 M EDTA, and cells were isolated by passing the digested tissue through a 70 μm filter (BD Biosciences) and rinsing with FACS buffer, PBS containing 0.5% Bovine Serum Albumin (BSA; Sigma) and 2 mM EDTA (Life Technologies). Red blood cells were lysed using ACK lysing buffer (Life Technologies). For analysis of tdTomato-positive tumour cells, samples were resuspended in FACS buffer and analysed using an LSR II flow cytometer (Becton Dickinson Immunocytometry Systems, BDIS). A standard curve was established for each organ by adding defined numbers of tumour cells into cells isolated from healthy lungs and livers and measuring the number of tdTomato-positive cells via flow cytometry. From this analysis, it was determined that the threshold tumour cell density of 0.002% (five tumour cells in 250,000 total cells) was consistently and significantly above background, and thus samples were deemed to have detectable cancer cells if the tumour cell density was above 0.002%. For analysis of leukocyte populations, cells were blocked with anti-CD16/32 (1:50, eBioscience) and stained for viability using fixable blue dead cell stain kit (Life Technologies). Cells were then stained with Alexa Fluor 700-conjugated anti-CD45 (30-F11, 1:125; Biolegend), Pacific Blue-conjugated anti-Gr-1 (RB6-8C5, 1:70; Biolegend), FITC-conjugated anti-Ly-6C (HK1.4, 1:100; Biolegend), PE-Cyanine7-conjugated anti-F4/80 (BM8, 1:70; Biolegend), APC-conjugated anti-CD11c (N418, 1:85; eBioscience), v500-conjugated anti-CD11b (M1/70, 1:100; BD Biosciences), Pacific Blue-conjugated anti-CD19 (6D5, 1:100; Biolegend), v500-conjugated anti-CD4 (RM4-5, 1:100; BD Biosciences), FITC-conjugated anti-CD8a (53-6.7, 1:25; Biolegend) and PE-Cyanine7-conjugated anti-CD49b (DX5, 1:40; Biolegend). Samples were analysed using an LSRFortessa flow cytometer (BDIS). Splenocyte isolation for transplants and media conditioning Spleens were isolated from tumour-bearing mice, minced using microscissors and incubated in a 0.38 mg ml −1 solution of Liberase TL (Roche Applied Science) for 20 min at 37 °C. The minced tissue was passed through a 70 μm strainer and red blood cells were lysed using ACK lysing buffer (Life Technologies). To collect Gr1 hi CD11b + cells, splenocytes were labelled with FITC-conjugated anti-Gr-1 (RB6-8C5, 1:100; Biolegend), APC-conjugated anti-Ly-6C (HK1.4, 1:50; Biolegend), and APC-eFluor780-conjugated anti-CD11b (M1/70, 1:100; eBioscience) and the Gr1 hi CD11b + Ly6C − population was collected via FACS sorting using a BD FACSAria cytometer (BDIS). The remaining splenocyte population (Gr1 hi CD11b + cell-depleted) was also collected. For cell transplantation studies, scaffolds were rinsed with RPMI medium (Life Technologies) containing 5% fetal bovine serum (FBS; Life Technologies) and dried on gauze. 1 × 10 6 Gr1 hi CD11b + cells were seeded on each scaffold in a volume of 5 μl RPMI with 5% FBS and scaffolds were implanted into the intraperitoneal fat pads. For generation of conditioned media, splenocytes, Gr1 hi CD11b + cells, and Gr1 hi CD11b + cell-depleted splenocytes were each plated at a concentration of 1 × 10 6 cells per ml in RPMI media. Media was conditioned for 48 h, after which the media was sterile-filtered to remove splenocytes. Splenocyte migration assays Migration assays were performed in 24-well transwell chambers with 5-μm pore size filters (Corning). A total of 1 × 10 6 splenocytes were placed in the top chamber in 100 μl of RPMI medium containing 10% FBS. 600 μl of RPMI medium containing 10% FBS with or without 100 ng ml −1 recombinant mouse CCL22 (Peprotech) was placed in the bottom chamber. After 1.5 h, the number of cells that had migrated to the bottom chamber was counted using a hemocytometer. Tumour cell migration assays Tumour cells were serum-starved overnight in DMEM (Sigma) or RPMI (Life Technologies) containing 0.2% FBS (Life technologies). Migration assays were performed in 24-well transwell chambers with 8-μm pore size filters (Corning). Total of 5 × 10 4 231BR or 4T1 cells were placed in the top chamber in 300 μl of DMEM (for CCL22 assays) or RPMI (for conditioned media assays) containing 0.2% FBS. For CCL22 assays, 750 μl of DMEM containing 0.2% FBS with or without 100 ng ml −1 recombinant human CCL22 or SDF1 (Peprotech) was placed in the bottom chamber. For conditioned media, 750 μl of RPMI, splenocyte-conditioned RPMI, Gr1 hi CD11b + cell-conditioned RPMI or RPMI conditioned with Gr1 hi CD11b + cell-depleted splenocytes was placed in the bottom chamber (all media was supplemented with 0.2% FBS). After 24 h, the cells on the top of the filter were removed by gently scrubbing with a cotton swab, and the cells on the bottom of the filter were stained for 60 min in a 0.5% ( w/v ) solution of crystal violet (Sigma) in 60% PBS/40% ethanol. The inserts were rinsed in PBS and the number of migrating cells was counted. Conditioning collagen gels with 231BR cells A 1.6 mg ml −1 collagen I solution was prepared by mixing rat tail Collagen I (BD Biosciences) with deionized water, 10 × PBS (Sigma, 1:10 dilution) and 1 N NaOH (Sigma, 1:1,000 dilution) on ice. Collagen solution (150 μl) was placed in each well of a 48-well plate. Gels were incubated at 37 °C for 1 h, after which 1.875 × 10 5 231BR cells in 400 μl of RPMI containing 10% FBS were seeded on each gel. Control gels received 400 μl of RPMI containing 10% FBS. After incubation at 37 °C for 3 days, cells were extracted from the gels. The media was removed from each well and the gels were washed three times with 1 × PBS (Life Technologies). A 20 mM NH 4 OH solution containing 0.5% (v/v) Triton X-100 (Sigma) was added to each well and the chamber slide was incubated at 37 °C for 5 min. After removal of the NH 4 OH/Triton X-100 solution, the gels were washed twice with distilled water and twice with PBS. A volume of 175 μl of PBS was added to each well before imaging. Scanning electron microscopy Structural characteristics of scaffolds were imaged with a scanning electron microscope (Hitachi s4800-II cFEG s.e.m. ; Hitachi High-Technologies Corp.). A 15-nm gold coating was applied and the microscope was operated at 2 kV. ISOCT imaging and analysis The OCT system used a Fourier domain configuration. A supercontinuum light source (NKT photonics, SuperK versa) provided a broadband laser from ∼ 500 to 840 nm. The spectral range from 650 to 830 nm was used for OCT image construction. The laser was delivered by an optical fibre, collimated by a lens, and input into a cube beam splitter (BS; Thorlabs, CM1-BS013), by which the light was divided into a sample arm and a reference arm. The reference arm consisted of a series of glass plates for dispersion control and a mirror reflecting the light backward. The sample arm consisted of a two-dimensional scanning mirror (Thorlabs, GVSM002) and an objective lens (effective numerical aperature=0.04; Zeiss) to focus the light on specimens. The lateral resolution is estimated as 15 μm. The interfered light from the reference and sample arm at the BS was collected by another optical fibre and delivered to the spectrometer for spectral acquisition. The mirror was scanning at a frequency of 2.56 kHz, and a 3D acquisition lasted 25.6 s with 256 by 256 pixels in two lateral directions. The camera exposure time was 0.3 ms. With the bandwidth, the axial resolution was estimated as 2 μm. The depth structural reconstruction was created by the following steps. The recorded spectrum was first normalized by the source spectrum, and then resampled into k domain with equal interval, and finally a Fourier transform was taken to recover the depth signal. k is the wave number, defined by k=2π/λ. The calculation of D value was performed by the following steps. A Gaussian window with width k w =0.36 μm −1 was applied on the spectrum, and the depth structural reconstruction process was performed. This process was then repeated with the Gaussian window scanning through the whole spectral range, and the wavelength-dependent 3D structure was obtained. The reduced range of spectrum relaxed the axial resolution to be about 20 μm. The averaged spectra from the specimen were modelled by I(k) = k 2-D/2 . The value of D was then obtained by calculating the power of the spectra. Statistical analysis Data are presented as mean±s.e.m., and P values were determined using a Mann–Whitney test for single comparisons. For comparison of relative numbers of mice containing metastasis to various tissues, a Fisher’s exact test was used to determine the P value. Statistical analysis was performed using GraphPad Prism. How to cite this article: Azarin, S. M. et al. In vivo capture and label-free detection of early metastatic cells. Nat. Commun. 6:8094 doi: 10.1038/ncomms9094 (2015).